Epsin is required for Dishevelled stability and Wnt signalling activation in colon cancer development Uncontrolled canonical Wnt signalling supports colon epithelial tumour expansion and malignant transformation. Understanding the regulatory mechanisms involved is crucial for elucidating the pathogenesis of and will provide new therapeutic targets for colon cancer. Epsins are ubiquitin-binding adaptor proteins upregulated in several human cancers; however, the involvement of epsins in colon cancer is unknown. Here we show that loss of intestinal epithelial epsins protects against colon cancer by significantly reducing the stability of the crucial Wnt signalling effector, dishevelled (Dvl2), and impairing Wnt signalling. Consistently, epsins and Dvl2 are correspondingly upregulated in colon cancer. Mechanistically, epsin binds Dvl2 via its epsin N-terminal homology domain and ubiquitin-interacting motifs and prohibits Dvl2 polyubiquitination and degradation. Our findings reveal an unconventional role for epsins in stabilizing Dvl2 and potentiating Wnt signalling in colon cancer cells to ensure robust colon cancer progression. The pro-carcinogenic role of Epsins suggests that they are potential therapeutic targets to combat colon cancer. Colon cancer is one of the most commonly diagnosed cancers in the United States and, although significant advances in early diagnosis and treatment have been made in the last several years, it remains a leading cause of cancer-related death (American Cancer Society). Future advances in the treatment of this disease depend heavily on a better understanding of the signalling cascades and molecular mechanisms involved in tumour development and progression. The canonical Wnt signalling cascade is known to play an important role in this process [1] , [2] . Under physiologic conditions, canonical Wnt signalling activation disassembles the Axin/glycogen synthase kinase 3 (GSK3)/adenomatous polyposis coli (APC) destruction complex, ultimately resulting in β-catenin stabilization and nuclear accumulation [3] , [4] , [5] , [6] , [7] . Nuclear β-catenin binds to and activates the T-cell factor (TCF)/lymphoid enhancer factor (LEF) transcription factors resulting in the expression of important cell proliferation factors, including cMyc and cyclin D1 (refs 8 , 9 , 10 , 11 ). Several mutations in Axin, GSK3, APC and β-catenin genes cause significant deregulated nuclear β-catenin accumulation, uncontrolled cell proliferation and malignant transformation in the colon epithelium [4] , [12] , [13] , [14] , [15] , [16] , [17] . In addition to deregulated nuclear β-catenin accumulation, other alterations in canonical Wnt signalling are also associated with cancer development such as the overexpression of several key upstream regulators including Wnt receptors (Frizzled (Fzd) and low-density lipoprotein receptor-related protein (LRP)) and cytoplasmic signalling adaptor, dishevelled (Dvl) [18] , [19] , [20] , [21] , [22] . Dvl is recruited to the heterodimeric Wnt receptor complex, consisting of a single Fzd and LRP, in response to ligand stimulation and plays a crucial role in mediating Axin/GSK3/APC destruction complex disassembly [23] , [24] . Given that both the Wnt receptors and Dvl are upregulated in cancer and result in elevated canonical Wnt signalling, it has been hypothesized that alterations in the stabilization and/or internalization of the Fzd:LRP:Dvl complex may contribute to the aberrant canonical Wnt signalling linked to colon cancer development [25] , [26] , [27] . Previous studies reported that Wnt signalling is activated by endocytosis [25] , [27] , [28] . In 2010, Dr Robertis’s group [26] demonstrated that Wnt-dependent internalization of the Fzd:LRP:Dvl complex is an important step in activating Wnt signalling; however, the regulatory mechanisms involved are still unknown. Our laboratory has a long-standing interest in the regulated internalization of cell surface receptors, specifically the role of epsins in this mechanism. We speculated that epsins may activate Wnt signalling by regulating Wnt-induced receptor complex endocytosis. Epsins are classically defined as clathrin-mediated endocytic adaptors that facilitate the internalization of ubiquitinated cell surface receptors [29] , [30] , [31] , [32] , [33] . Mammals express three highly conserved epsins: epsins 1 and 2, which are ubiquitously expressed in most cell types, and epsin 3, which is primarily expressed in the skin and stomach [30] , [31] , [34] , [35] , [36] . Epsins 1 and 2 are redundant in function as indicated by the fact that mice lacking either epsin 1 or 2 survive normally with no obvious phenotypic alterations, while mice lacking both epsins 1 and 2 die in utero [34] . In order to bypass embryonic lethality, we previously generated a conditional epsin 1 mouse on an epsin 2 null background [37] . Importantly, these mice, which undergo post-developmental epsin 1 deletion, survive normally under physiologic conditions. Interestingly, we recently reported that under pathological conditions, such as cancer, loss of endothelial epsins altered tumour angiogenesis resulting in reduced tumour growth and progression [37] , [38] . In addition to playing a role in regulating the tumour microenvironment, epsins are upregulated in skin, mammary and prostate tumours [36] , [39] , [40] , [41] . However, whether and how epsins promote colon cancer development are important and open questions. In this study, we investigate the potential role that epsins play in regulating colon cancer development using a unique colon cancer mouse model with inducible intestinal epithelial cell (IEpC)-specific epsin deficiency. We discover that epsin deficiency impairs canonical Wnt signalling and results in a colon cancer-resistant phenotype. Surprisingly, mechanistic analyses reveal that epsins are dispensable for the Wnt-induced endocytosis of receptors. Instead, epsins constitutively interact with and protect Dvl2 from polyubiquitination and proteasomal degradation, making them an essential regulator of Dvl2 stability. Without epsins, the Dvl2 protein pool is diminished, thus preventing downstream canonical Wnt signalling activation. This novel role for epsins as a critical chaperone protein is completely unexpected. Because Dvl2 is reportedly upregulated in and contributes to cancer progression [19] , [21] , [22] , we propose a model in which epsin upregulation during the early stages of tumorigenesis promotes Dvl2 stabilization, deregulates canonical Wnt signalling and facilitates colon cancer development [21] , [22] . Epsins are upregulated in human colon cancer We previously established that epsins play an important oncogenic role in regulating tumour microenvironments [37] ; however, whether epsins played a specific role in promoting tumour cell transformation and proliferation was largely unknown. Using an Oncomine database from The National Cancer Institute Cancer Genome Atlas containing publically available cDNA microarray data, we found that the gene expression of epsin 1 and epsin 2 was significantly upregulated in human colon cancer ( Fig. 1a,b ). Given that epsin 1 gene expression was significantly higher than epsin 2 in the HT-29 human colorectal adenocarcinoma cell line ( Fig. 1c ) [14] , [42] , we used immunofluorescence (IF) to analyse epsin 1 protein in human tissue microarrays containing colon adenomas, adenocarcinomas and corresponding non-neoplastic tissues ( Fig. 1d ). Epsin 1 upregulation correlated strongly with increased colon cancer severity ( Fig. 1d,e ) [43] . Epsin 1 upregulation also correlated strongly with increased levels of the Wnt receptor, Fzd7 ( Fig. 1d,f ), and downstream effector, Dvl2 ( Fig. 1d,g ). 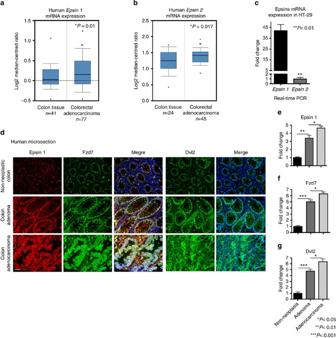Figure 1: Epsins were augmented in human colon cancer. (a,b) Humanepsin 1(a) andepsin 2(b) mRNA expression levels in normal colon and colorectal adenocarcinoma tissues. Data were retrieved from National Cancer Institute The Cancer Genome Atlas (TCGA) Oncomine data set. (c) qRT–PCR analysis ofepsin 1andepsin 2mRNA expression in HT-29 human colon cancer cells,n=9. (d) Representative immunofluorescence images of epsin 1, Fzd7 and Dvl2 in peripheral non-neoplastic, adenoma and adenocarcinoma colon tissues from an AccuMax human tissue microarray. Scale bar, 50 μM. (e–g) Quantification ofd,n=12. All statistical values were calculated using a Student’st-test;Pvalues are indicated. Error bars indicate the mean±s.e.m. Figure 1: Epsins were augmented in human colon cancer. ( a , b ) Human epsin 1 ( a ) and epsin 2 ( b ) mRNA expression levels in normal colon and colorectal adenocarcinoma tissues. Data were retrieved from National Cancer Institute The Cancer Genome Atlas (TCGA) Oncomine data set. ( c ) qRT–PCR analysis of ep sin 1 and epsin 2 mRNA expression in HT-29 human colon cancer cells, n =9. ( d ) Representative immunofluorescence images of epsin 1, Fzd7 and Dvl2 in peripheral non-neoplastic, adenoma and adenocarcinoma colon tissues from an AccuMax human tissue microarray. Scale bar, 50 μM. ( e – g ) Quantification of d , n =12. All statistical values were calculated using a Student’s t -test; P values are indicated. Error bars indicate the mean±s.e.m. Full size image Intestinal epithelial epsin loss prohibits colon cancer Encouraged by the upregulation of epsins in human colon cancer, we hypothesized that epsins, specifically intestinal epithelial epsins, may play a crucial role in propagating colon cancer cell transformation and/or proliferation. To test this, we generated a novel mouse model selectively lacking epsin 1 in IEpCs on an epsin 2 null background by crossing Epn1 fl/fl ;Epn2 −/− mice [34] , [37] with mice expressing tamoxifen-inducible Cre recombinase under control of the Villin promoter ( Villin-ER T2 Cre ) [44] . To produce inducible IEpC-iDKO (double knockout) mice, gender and genetic background-matched 10-week-old wild-type (WT) or Epn1 fl/fl ;Epn2 −/− ; Villin-ER T2 Cre mice were intraperitoneally injected with tamoxifen every second day for 2 weeks. Deletion of epsins 1 and 2 in the colon of IEpC-iDKO mice was validated by western blotting ( Fig. 2a,b ). 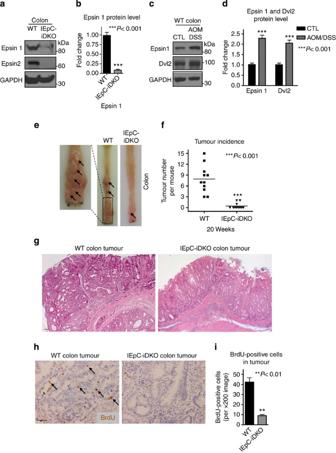Figure 2: Intestinal epithelial epsin deficiency reduced tumour growth in a colon cancer mouse model. (a) Western blotting of epsins 1 and 2 in colon epitheliums from WT and IEpC-iDKO mice. (b) Quantification ofa,n=6. (c) Western blotting of epsin 1 and Dvl2 in colon epithelia from control (CTL) and AOM/DSS-treated WT mice. (d) Quantification ofc,n=6. (e) Longitudinally cut colons and rectums of WT and IEpC-iDKO mice killed 20 weeks post-AOM/DSS treatment; arrows indicate tumours in the colon and rectal regions. (f) Quantification of tumour incidence ine,n=11. (g) H&E staining from representative WT and IEpC-iDKO colons frome,n=11; × 10 objective. Scale bar, 50 μm. (h)In vivoBrdU immunohistochemistry of WT and IEpC-iDKO colons 20 weeks post-AOM/DSS treatment; × 20 objective; arrows indicate BrdU-positive cells. Scale bar, 50 μm. (i) Quantification of BrdU immunohistochemistry inh,n=11. All statistical values were calculated using a Student’st-test;Pvalues are indicated. Error bars indicate the mean±s.e.m. Figure 2: Intestinal epithelial epsin deficiency reduced tumour growth in a colon cancer mouse model. ( a ) Western blotting of epsins 1 and 2 in colon epitheliums from WT and IEpC-iDKO mice. ( b ) Quantification of a , n =6. ( c ) Western blotting of epsin 1 and Dvl2 in colon epithelia from control (CTL) and AOM/DSS-treated WT mice. ( d ) Quantification of c , n =6. ( e ) Longitudinally cut colons and rectums of WT and IEpC-iDKO mice killed 20 weeks post-AOM/DSS treatment; arrows indicate tumours in the colon and rectal regions. ( f ) Quantification of tumour incidence in e , n =11. ( g ) H&E staining from representative WT and IEpC-iDKO colons from e , n =11; × 10 objective. Scale bar, 50 μm. ( h ) In vivo BrdU immunohistochemistry of WT and IEpC-iDKO colons 20 weeks post-AOM/DSS treatment; × 20 objective; arrows indicate BrdU-positive cells. Scale bar, 50 μm. ( i ) Quantification of BrdU immunohistochemistry in h , n =11. All statistical values were calculated using a Student’s t -test; P values are indicated. Error bars indicate the mean±s.e.m. Full size image We utilized the IEpC-iDKO mice in an azoxymethane/dextran sulfate sodium (AOM/DSS)-induced colon cancer model to investigate the role of epsins in colon cancer development [45] , [46] . Similar to human colon cancer, AOM/DSS-induced colon cancer in WT mice 20 weeks post treatment exhibited significantly increased epsin 1 and Dvl2 protein levels ( Fig. 2c,d ), indicative of epsins having a potential pro-carcinogenic role. In contrast, loss of epsins in the IEpC-iDKO colons revealed a striking tumour-resistant phenotype with significantly fewer tumours, indicated by arrows ( Fig. 2e,f ). haematoxylin and eosine (H&E) staining of isolated colons revealed only moderately differentiated adenomas in IEpC-iDKO mice but typical tubular adenocarcinomas with metastasis across the basement membrane in WT mice ( Fig. 2g ) [43] . We used in vivo bromodeoxyuridine (BrdU) labelling and immunohistochemical (IHC) staining to determine whether the tumour-resistant phenotype in IEpC-iDKO colons resulted from impaired colon epithelial tumour cell proliferation. We found that IEpC-iDKO colons incorporated significantly less BrdU, indicated by arrows ( Fig. 2h,i ). Collectively, these data showed that specific loss of epsins in the colon epithelium hindered tumour cell proliferation and colon cancer progression in vivo . Canonical Wnt signalling is impaired in IEpC-iDKO mice We hypothesized that loss of colon epithelial epsins protected against colon cancer by interfering with the aberrant canonical Wnt signalling associated with human colon cancer [1] , [2] , [47] . First, we measured nuclear β-catenin accumulation, the hallmark of canonical Wnt signalling, in colon tumours isolated from WT and IEpC-iDKO mice. WT colon tumours exhibited heavy nuclear β-catenin staining, as indicated by its colocalization with the nuclear haematoxylin stain, while the moderately differentiated IEpC-iDKO colon tumours exhibited very little staining ( Fig. 3a ). Western blotting confirmed that colon epithelial epsin deficiency significantly hindered β-catenin accumulation ( Fig. 3b,c ). Accumulated β-catenin transports to the nucleus where it binds to and activates the TCF/LEF transcription factors resulting in the expression of cMyc and cyclin D1 (refs 8 , 9 , 10 ). Using quantitative real-time PCR (qRT–PCR), we confirmed that the IEpC-iDKO colon epithelium exhibited significant deficiencies in both cMyc and cyclin D1 mRNA expression ( Fig. 3d ). In summary, our in vivo data strongly indicated that epsin loss protected against colon cancer development by hindering aberrant canonical Wnt signalling. 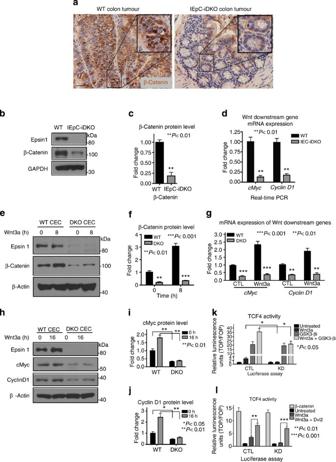Figure 3: Epsin deficiency significantly inhibited downstream canonical Wnt signalling. (a) β-Catenin immunohistochemistry of WT or IEpC-iDKO colon tumours isolated 20 weeks post-AOM/DSS treatment; × 20 objective. Scale bar, 50 μM,n=11. (b–d) Lysates from isolated colon epithelia of adult WT and IEpC-iDKO mice analysed by western blotting for epsin 1 deletion and β-catenin protein accumulation (b,c) or by qRT–PCR forcMycandcyclin D1mRNA expression (d),n=9. (e,f) Primary WT and epsins 1 and 2 DKO CECs isolated and cultured from WT or IEpC-iDKO pups, respectively, and then stimulated with Wnt3a (100 ng ml−1) for 8 h were analysed by western blotting for β-catenin,n=8. (g) CECs treated with Wnt3a for 12 h were analysed by qRT–PCR forcMycandcyclin D1mRNA expression,n=9. (h–j) CECs treated with Wnt3a for 16 h were analysed by western blotting for cMyc and cyclin D1,n=8. (k,l) β-Catenin-dependent TCF4 transcriptional activation in response to Wnt3a stimulation without or with the GSK3 inhibitor, GSK3-βi, (k) or in the presence of unphosphorylatable β-catenin (β-catenin) or Dvl2 (l) was measured in CTL or epsins 1 and 2 KD HEK 293T cells transfected with TOPflash or FOPflash luciferase expression vectors and Renilla,n=8. All statistical values were calculated using a Student’st-test;Pvalues are indicated. Error bars indicate the mean±s.e.m. Figure 3: Epsin deficiency significantly inhibited downstream canonical Wnt signalling. ( a ) β-Catenin immunohistochemistry of WT or IEpC-iDKO colon tumours isolated 20 weeks post-AOM/DSS treatment; × 20 objective. Scale bar, 50 μM, n =11. ( b – d ) Lysates from isolated colon epithelia of adult WT and IEpC-iDKO mice analysed by western blotting for epsin 1 deletion and β-catenin protein accumulation ( b , c ) or by qRT–PCR for cMyc and cyclin D1 mRNA expression ( d ), n =9. ( e , f ) Primary WT and epsins 1 and 2 DKO CECs isolated and cultured from WT or IEpC-iDKO pups, respectively, and then stimulated with Wnt3a (100 ng ml − 1 ) for 8 h were analysed by western blotting for β-catenin, n =8. ( g ) CECs treated with Wnt3a for 12 h were analysed by qRT–PCR for cMyc and cyclin D1 mRNA expression, n =9. ( h – j ) CECs treated with Wnt3a for 16 h were analysed by western blotting for cMyc and cyclin D1, n =8. ( k , l ) β-Catenin-dependent TCF4 transcriptional activation in response to Wnt3a stimulation without or with the GSK3 inhibitor, GSK3-βi, ( k ) or in the presence of unphosphorylatable β-catenin (β-catenin) or Dvl2 ( l ) was measured in CTL or epsins 1 and 2 KD HEK 293T cells transfected with TOPflash or FOPflash luciferase expression vectors and Renilla, n =8. All statistical values were calculated using a Student’s t -test; P values are indicated. Error bars indicate the mean±s.e.m. Full size image Canonical Wnt signalling is attenuated in colon cancer cells To understand the mechanism(s) by which increased epsin expression promoted colon epithelial cell (CEC) transformation and colon tumour proliferation, it was important to first understand the physiologic role of epsins. Towards this end, we isolated and cultured primary CECs from WT and Epn1 fl/fl ;Epn2 −/− ; Villin-ER T2 Cre pups. Epsin 1 deletion was induced ex vivo by tamoxifen-treatment (DKO CEC) and was confirmed by western blotting ( Fig. 3e ). Consistent with our in vivo findings, DKO CECs exhibited significantly less β-catenin stabilization ( Fig. 3e,f ) and downstream target gene expression ( Fig. 3g–j ) compared with WT CECs. Importantly, epsin deficiency significantly reduced β-catenin accumulation and transcriptional activation independent of Wnt stimulation ( Fig. 3e–j ), suggesting that the loss of epsins hindered canonical Wnt signalling upstream of β-catenin stabilization. To test this, we employed a luciferase assay using the β-catenin-dependent TOPflash reporter as readout of TCF4 activity. Before lysis, control and short interfering RNA (siRNA)-mediated epsin-deficient (KD; knockdown) HEK 293T cells transfected with the luciferase vector system were treated without or with a GSK3-β inhibitor, GSK3-βi, and Wnt3a. As expected, loss of epsins significantly impaired Wnt-mediated TCF4 transcriptional activation ( Fig. 3k,l ); however, GSK3-βi treatment, which disassembled the β-catenin destruction complex, significantly increased TCF4 transcriptional activity in both control and KD cells under resting condition ( Fig. 3k ). Importantly, while Wnt stimulation further increased TCF4 transcriptional activity in GSK3-βi-treated control cells, it failed to do so in KD cells, thus suggesting epsins regulated Wnt-dependent signalling upstream of the destruction complex. Consistently, overexpression of constitutively active unphosphorylatable β-catenin produced maximal transcriptional activity in both control and KD cells regardless of stimulation ( Fig. 3l ). Further, overexpression of Wnt receptor effector, Dvl2, rescued Wnt-dependent signalling in KD cells, supporting that the action of epsin-mediated regulation of Wnt signalling is at the receptor level ( Fig. 3l ). Wnt-receptor endocytosis is independent of epsins Given the classic role of epsin as an endocytic adaptor protein and that Wnt signalling is reportedly activated by receptor internalization [25] , [26] , [27] , [28] , [30] , [31] , [48] , we originally hypothesized that epsins might potentiate Wnt signalling by facilitating Wnt receptor endocytosis. To determine whether epsin interacted with Wnt receptors endogenously, we performed co-immunoprecipitation assays in HT-29 cells using an epsin 1-specific antibody. We found that endogenous epsin 1 bound endogenous Wnt receptors, Fzd7 and LRP6, in a Wnt-dependent manner ( Fig. 4a,b )—a finding consistent with Wnt-dependent recruitment of epsin 1 to the Wnt receptor complex. Epsin loss also significantly hindered Wnt-dependent LRP6 phosphorylation in CECs ( Fig. 4c,d ), further suggesting impaired Wnt signalling activation. Given the cumulative evidence supporting a role for epsins in regulating Wnt receptor internalization and activation, we were surprised to find that loss of epsins failed to impair Wnt-mediated LRP6 internalization in CECs ( Fig. 4e,f ). Briefly, we used a cleavable biotinylation kit to label receptors on the surface of chilled WT and DKO CECs. CECs were washed with warm media, stimulated for various times with Wnt3a and then chilled again; any remaining biotinylation on the surface was cleaved. Internalized biotin-labelled receptors were immunoprecipitated with streptavidin and analysed by western blotting using a LRP6-specific antibody. LRP6 was internalized with similar efficiency after 5 min of Wnt stimulation in both WT and DKO CECs ( Fig. 4e,f ), suggesting that Wnt-dependent internalization of the Wnt receptor complex was not regulated by or dependent on epsin. 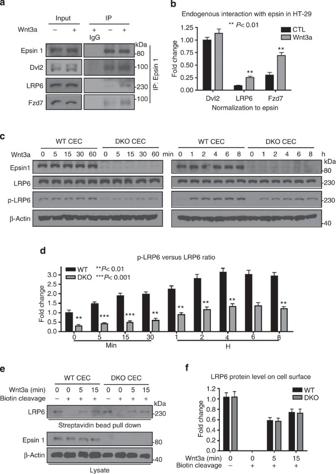Figure 4: Epsin interacted with Dvl2 to regulate Wnt receptor signalling independent of receptor-mediated endocytosis. (a) Co-immunoprecipitation of endogenous Dvl2, LRP6 and Fzd7 by anti-epsin 1 antibody in Wnt3a-stimulated (100 ng ml−1, 5 min) HT-29 cells analysed by western blotting. (b) Quantification ofa,n=8. (c) WT and DKO CECs were stimulated with Wnt3a (100 ng ml−1) as indicated then Wnt signalling was analysed by western blotting with LRP6 and phospho-LRP6 antibodies. (d) Quantification of phospho-to-total LRP6 fold change inc,n=8. (e) Cell surface of WT and DKO CECs were labelled with cleavable biotin, incubated with Wnt3a at 37 °C as indicated and then the surface biotin was cleaved. Internalized biotinylated LRP6 was determined by streptavidin bead pull-down and Western blotting. (f) Quantification ofe,n=8. All statistical values were calculated using a Student’st-test;Pvalues are indicated. Error bars indicate the mean±s.e.m. Figure 4: Epsin interacted with Dvl2 to regulate Wnt receptor signalling independent of receptor-mediated endocytosis. ( a ) Co-immunoprecipitation of endogenous Dvl2, LRP6 and Fzd7 by anti-epsin 1 antibody in Wnt3a-stimulated (100 ng ml − 1 , 5 min) HT-29 cells analysed by western blotting. ( b ) Quantification of a , n =8. ( c ) WT and DKO CECs were stimulated with Wnt3a (100 ng ml − 1 ) as indicated then Wnt signalling was analysed by western blotting with LRP6 and phospho-LRP6 antibodies. ( d ) Quantification of phospho-to-total LRP6 fold change in c , n =8. ( e ) Cell surface of WT and DKO CECs were labelled with cleavable biotin, incubated with Wnt3a at 37 °C as indicated and then the surface biotin was cleaved. Internalized biotinylated LRP6 was determined by streptavidin bead pull-down and Western blotting. ( f ) Quantification of e , n =8. All statistical values were calculated using a Student’s t -test; P values are indicated. Error bars indicate the mean±s.e.m. Full size image How then was epsin regulating the activation of canonical Wnt signalling? To answer this, we returned to our co-immunoprecipitation assay and found that endogenous epsin 1 constitutively interacted with the crucial cytoplasmic signalling effector, Dvl2, independent of Wnt stimulation ( Fig. 4a,b ). Notably, Dvl2 was not immunoprecipitated in epsin-deficient HT-29 cells, indicating the specificity of the epsin:Dvl2 interaction ( Supplementary Fig. 1 ). Dvl interacts with the cytoplasmic tail of LRP in response to Wnt stimulation and plays a crucial role in the recruitment, phosphorylation and disassembly of the β-catenin destruction complex [6] , [23] , [24] , [49] . In light of this new finding, we hypothesized that epsins interacted with and stabilized Dvl2, thus protecting it from degradation to ensure Wnt signalling activation. Epsin regulates Dvl2 stability To test the hypothesis that epsins regulated Dvl2 stability, we used western blotting to determine whether the loss of epsins would reduce total Dvl2 protein. Given that Dvl2 overexpression is strongly associated with colon cancer [19] , [22] , a result we confirmed using qRT–PCR of the CMT-93 mouse colon cancer cell line compared with WT CECs ( Fig. 5c ), we focused our attention on the relationship between epsins and Dvl2. We found that epsin deficiency, either in DKO CECs ( Fig. 5a,b ) or in siRNA-mediated KD in HT-29 cells ( Fig. 5d,e ), significantly reduced total Dvl2 protein levels. Importantly, epsin loss did not hinder Wnt-dependent Dvl2 phosphorylation as indicated by the molecular weight shift in the western blotting ( Fig. 5a,b,d,e ). Further, loss of epsins did not alter mRNA expression of Dvl1 , Dvl2 or Dvl3 in CECs ( Fig. 5f ), suggesting that loss of the Dvl2 protein was due to increased degradation and not due to decreased transcription. To confirm, we treated WT CECs with the proteasomal inhibitor, MG132, to impair Dvl2 degradation. Surprisingly, MG132 treatment significantly increased both epsin 1 and Dvl2 protein levels ( Fig. 5g–i ) without altering gene expression ( Fig. 5j,k ). These results demonstrated that epsin 1 and Dvl2 can be degraded via the proteasome and indicated a correlation between epsin 1 protein levels and Dvl2 stability. To confirm that Dvl2 protein levels were directly regulated by epsin 1, we created a gradient of epsin 1 depletions in the epsin 2 null CECs by adjusting tamoxifen exposure and measured Dvl2 protein levels. We found that greater loss of endogenous epsin 1 resulted in greater loss of endogenous Dvl2 ( Fig. 5l ). Cumulatively, these data uncovered a novel role for epsins in the stabilization of Dvl2 and Wnt signalling. 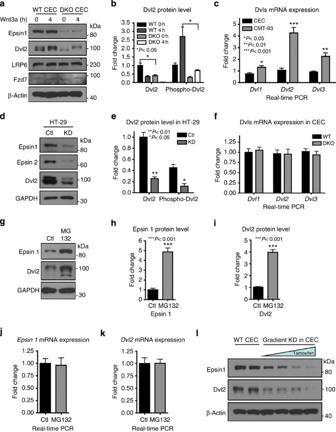Figure 5: Epsin interacted with and stabilized Dvl2 to promote Wnt signalling. (a) CECs were stimulated with Wnt3a (100 ng ml−1) for 4 h, and then endogenous epsin 1, Dvl2, LRP6 and Fzd7 proteins were analysed by western blotting. (b) Quantification of total and phospho-Dvl2 ina,n=8. (c) qRT–PCR analyses ofDvl1,Dvl2andDvl3mRNA expressions in WT CECs and the CMT-93 mouse colon cancer cell line,n=9. (d) Western blotting of epsins 1 and 2 and Dvl2 in CTL and siRNA-mediated epsin-deficient (KD) HT-29 human colon cancer cells. (e) Quantification of total and phospho-Dvl2 ind,n=8. (f) qRT–PCR analyses ofDvl1,Dvl2andDvl3mRNA expressions in WT and DKO CECs,n=9. (g) Western blotting of epsin 1 and Dvl2 in WT CECs after 4-h treatment with 10 μM proteasomal inhibitor, MG132. (h,i) Quantifications of epsin 1 (h) and Dvl2 (i) ing,n=8. (j,k) qRT–PCR analyses ofepsin 1(j) andDvl2(k) mRNA expressions in WT CECs after the MG132 treatment,n=9. (l) Western blotting of epsin 1 and Dvl2 in CECs with a variable tamoxifen-induced gradient of epsin 1 KD,n=8. All statistical values were calculated using a Student’st-test;Pvalues are indicated. Error bars indicate the mean±s.e.m. Figure 5: Epsin interacted with and stabilized Dvl2 to promote Wnt signalling. ( a ) CECs were stimulated with Wnt3a (100 ng ml − 1 ) for 4 h, and then endogenous epsin 1, Dvl2, LRP6 and Fzd7 proteins were analysed by western blotting. ( b ) Quantification of total and phospho-Dvl2 in a , n =8. ( c ) qRT–PCR analyses of Dvl1 , Dvl2 and Dvl3 mRNA expressions in WT CECs and the CMT-93 mouse colon cancer cell line, n =9. ( d ) Western blotting of epsins 1 and 2 and Dvl2 in CTL and siRNA-mediated epsin-deficient (KD) HT-29 human colon cancer cells. ( e ) Quantification of total and phospho-Dvl2 in d , n =8. ( f ) qRT–PCR analyses of Dvl1 , Dvl2 and Dvl3 mRNA expressions in WT and DKO CECs, n =9. ( g ) Western blotting of epsin 1 and Dvl2 in WT CECs after 4-h treatment with 10 μM proteasomal inhibitor, MG132. ( h , i ) Quantifications of epsin 1 ( h ) and Dvl2 ( i ) in g , n =8. ( j , k ) qRT–PCR analyses of epsin 1 ( j ) and Dvl2 ( k ) mRNA expressions in WT CECs after the MG132 treatment, n =9. ( l ) Western blotting of epsin 1 and Dvl2 in CECs with a variable tamoxifen-induced gradient of epsin 1 KD, n =8. All statistical values were calculated using a Student’s t -test; P values are indicated. Error bars indicate the mean±s.e.m. Full size image Epsin ENTH and UIM domains interact with Dvl2 Epsins are multidomain proteins with the most notable domains being the two highly conserved ubiquitin-interacting motifs (UIM) responsible for epsin interaction with ubiquitinated cell surface receptors [29] , [32] , [37] , [50] , [51] , [52] . Given that proteasomal degradation of proteins such as Dvl2 is dependent on polyubiquitination [53] , we hypothesized that the epsin:Dvl2 interaction may be facilitated by epsin UIM binding to polyubiquitinated Dvl2. To determine whether the epsin UIM was responsible for the epsin:Dvl2 interaction, we co-immunoprecipitated Dvl2 using either full-length epsin 1 or an epsin 1 construct lacking the UIM region (epsin 1 ΔUIM) and found that the epsin 1 ΔUIM only partially inhibited the interaction between epsin 1 and Dvl2 suggesting that, while it does play a role, the UIM was not sufficient to mediate epsin:Dvl2 interaction ( Fig. 6a ; Supplementary Fig. 2a ). Interestingly, the UIM did mediate the Wnt-dependent interaction between epsin 1 and the Wnt receptors ( Supplementary Fig. 2b–d ), a finding that suggests a multifaceted nature for epsin, and its UIM domain, in canonical Wnt signalling. 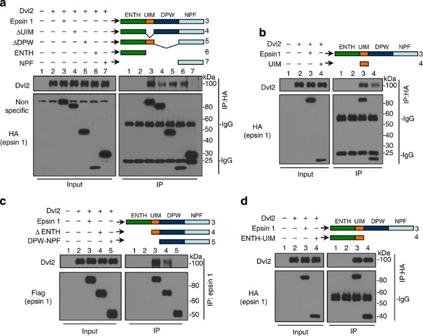Figure 6: Epsin 1 interacted with Dvl2 via its ENTH and UIM domains. Epsin 1 full-length (Epsin 1) and the following truncated epsin 1 constructs were co-transfected with full-length Dvl2 into HEK 293T cells: HA-tagged full-length epsin 1 (Epsin 1) (a,b,d), Epsin 1 ΔUIM (ΔUIM) (a), Epsin 1 ΔDPW (ΔDPW) (a), ENTH alone (ENTH) (a), NPF alone (NPF) (a), UIM alone (UIM) (b) and ENTH-UIM alone (ENTH-UIM) (d); Flag-tagged Epsin 1 full-length (Epsin 1;c), Epsin 1 ΔENTH (ΔENTH;c) and DPW-NPF alone (DPW-NPF) (c). (a–d) Dvl2 was co-immunoprecipitated by specified epsin 1 constructs using anti-HA (a,b,d) or anti-epsin 1 (c) antibodies, and then analysed by western blotting. All are representative blots fromn=8. Figure 6: Epsin 1 interacted with Dvl2 via its ENTH and UIM domains. Epsin 1 full-length (Epsin 1) and the following truncated epsin 1 constructs were co-transfected with full-length Dvl2 into HEK 293T cells: HA-tagged full-length epsin 1 (Epsin 1) ( a , b , d ), Epsin 1 ΔUIM (ΔUIM) ( a ), Epsin 1 ΔDPW (ΔDPW) ( a ), ENTH alone (ENTH) ( a ), NPF alone (NPF) ( a ), UIM alone (UIM) ( b ) and ENTH-UIM alone (ENTH-UIM) ( d ); Flag-tagged Epsin 1 full-length (Epsin 1; c ), Epsin 1 ΔENTH (ΔENTH; c ) and DPW-NPF alone (DPW-NPF) ( c ). ( a – d ) Dvl2 was co-immunoprecipitated by specified epsin 1 constructs using anti-HA ( a , b , d ) or anti-epsin 1 ( c ) antibodies, and then analysed by western blotting. All are representative blots from n =8. Full size image Epsin contains several other potential binding domains that may work in combination with the UIM to efficiently interact with and protect Dvl2 including the epsin N-terminal homology (ENTH), DPW and NPF domains [29] , [30] , [51] . To determine the role that these domains play in the epsin:Dvl2 interaction, we utilized epsin 1 truncation constructs lacking the ENTH domain (epsin 1 ΔENTH) or DPW motif (epsin 1 ΔDPW) or containing a single binding domain (ENTH, UIM or NPF) to co-immunoprecipitate Dvl2. We found that ENTH alone ( Fig. 6a ) and UIM alone ( Fig. 6b ) or constructs containing ENTH (ΔUIM and ΔDPW ( Fig. 6a )) or UIM (ΔDPW ( Fig. 6a ) and ΔENTH ( Fig. 6c )) all partially immunoprecipitated Dvl2. In contrast, neither NPF alone ( Fig. 6a ) nor DPW-NPF ( Fig. 6c ) interacted with Dvl2. From these binding data, we proposed that epsin interacted constitutively with Dvl2 through cooperative binding by the ENTH and UIM domains, a hypothesis supported by the fact that an ENTH-UIM construct was the only one tested that co-immunoprecipitated Dvl2 comparably to full-length epsin 1 ( Fig. 6d ). Dvl2 ubiquitination is reduced by Epsin ENTH-UIM binding It is well established that Dvl2 polyubiquitination is facilitated by the interaction of the Dvl2 C terminus with various E3 ligases [53] , [54] , [55] , [56] , [57] . We hypothesized that epsin may protect Dvl2 from degradation by competitively interfering with E3 ligase binding at the C terminus of Dvl2. To test this and map the epsin 1-binding domains within Dvl2, we generated Dvl2 truncation constructs containing either the N-terminal DIX and PDZ domains (DIX-PDZ) or C-terminal DEP and YHEL domains (DEP-YHEL). Only Dvl2 constructs containing the C-terminal DEP and YHEL domains were polyubiquitinated ( Fig. 7a ). Epsin 1 interacted with and co-immunoprecipitated full-length Dvl2 and the DEP-YHEL construct but failed to interact with the DIX-PDZ construct ( Fig. 7b ). Reciprocally, Dvl2 lacking only the DIX domain (ΔDIX) was sufficient to immunoprecipitate epsin 1 comparably, if not more efficiently, than full-length Dvl2 ( Fig. 7c ). Collectively, our binding studies suggested that the N-terminal ENTH-UIM domain of epsin interacted with the C-terminal domains of Dvl2. 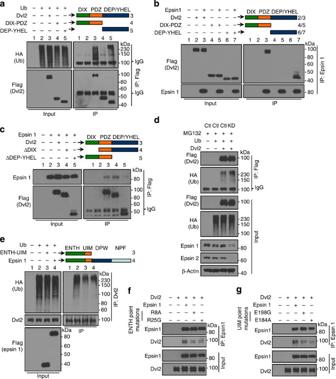Figure 7: Epsin ENTH-UIM interacted with and impaired polyubiquitination of the Dvl2 C terminus. (a) Polyubiquitinated full-length or truncated flag-tagged Dvl2 was immunoprecipitated using anti-flag antibody in HEK 293T cells transfected with Flag-tagged Dvl2 full-length (Dvl2), DIX-PDZ alone (DIX-PDZ) or DEP-YHEL alone (DEP-YHEL) constructs and HA-tagged ubiquitin and then analysed by western blotting. (b) Specified flag-tagged Dvl2 constructs were co-immunoprecipitated using anti-epsin 1 antibody in HEK 293T cells transfected with specified flag-tagged Dvl2 constructs and full-length epsin 1 and then were analysed by western blotting. (c) Epsin 1 was co-immunoprecipitated using anti-flag antibody in HEK 293T cells transfected with Flag-tagged Dvl2 full-length (Dvl2), Dvl2 ΔDIX (ΔDIX) or Dvl2 ΔDEP-YHEL (ΔDEP-YHEL) constructs and full-length epsin 1 and then were analysed by western blotting. (d) Polyubiquitinated full-length flag-tagged Dvl2 was immunoprecipitated using anti-flag antibody in MG132-treated CTL or epsins 1 and 2 KD HEK 293T cells transfected with flag-tagged Dvl2 and HA-tagged ubiquitin and then were analysed by western blotting. (e) Polyubiquitinated endogenous Dvl2 was immunoprecipitated using anti-Dvl2 antibody in HEK 293T cells transfected with specified flag-tagged epsin 1 constructs and HA-tagged ubiquitin and then were analysed by western blotting. (f,g) Dvl2 was co-immunoprecipitated using anti-epsin 1 antibody in HEK 293T cells transfected with specified mutant epsin 1 constructs and Dvl2 and then were analysed by western blotting. All are representative blots fromn=8. Figure 7: Epsin ENTH-UIM interacted with and impaired polyubiquitination of the Dvl2 C terminus. ( a ) Polyubiquitinated full-length or truncated flag-tagged Dvl2 was immunoprecipitated using anti-flag antibody in HEK 293T cells transfected with Flag-tagged Dvl2 full-length (Dvl2), DIX-PDZ alone (DIX-PDZ) or DEP-YHEL alone (DEP-YHEL) constructs and HA-tagged ubiquitin and then analysed by western blotting. ( b ) Specified flag-tagged Dvl2 constructs were co-immunoprecipitated using anti-epsin 1 antibody in HEK 293T cells transfected with specified flag-tagged Dvl2 constructs and full-length epsin 1 and then were analysed by western blotting. ( c ) Epsin 1 was co-immunoprecipitated using anti-flag antibody in HEK 293T cells transfected with Flag-tagged Dvl2 full-length (Dvl2), Dvl2 ΔDIX (ΔDIX) or Dvl2 ΔDEP-YHEL (ΔDEP-YHEL) constructs and full-length epsin 1 and then were analysed by western blotting. ( d ) Polyubiquitinated full-length flag-tagged Dvl2 was immunoprecipitated using anti-flag antibody in MG132-treated CTL or epsins 1 and 2 KD HEK 293T cells transfected with flag-tagged Dvl2 and HA-tagged ubiquitin and then were analysed by western blotting. ( e ) Polyubiquitinated endogenous Dvl2 was immunoprecipitated using anti-Dvl2 antibody in HEK 293T cells transfected with specified flag-tagged epsin 1 constructs and HA-tagged ubiquitin and then were analysed by western blotting. ( f , g ) Dvl2 was co-immunoprecipitated using anti-epsin 1 antibody in HEK 293T cells transfected with specified mutant epsin 1 constructs and Dvl2 and then were analysed by western blotting. All are representative blots from n =8. Full size image To capture the polyubiquitinated state of Dvl2, we treated HEK 293T cells overexpressing Dvl2 and haemagglutinin (HA)-tagged ubiquitin with MG132, then lysed the cells, immunoprecipitated Dvl2 and analysed Dvl2 ubiquitination by western blotting. Consistent with previous reports, Dvl2 was constitutively polyubiquitinated ( Fig. 7d ). Notably, epsin depletion increased Dvl2 polyubiquitination after MG132 treatment. To determine whether epsin ENTH-UIM could protect Dvl2 from polyubiquitination, we overexpressed full-length epsin 1 or ENTH-UIM in combination with HA-tagged ubiquitin and measured the endogenous Dvl2 ubiquitination status. Consistent with the epsin:Dvl2 interaction interfering with E3 ligase binding to Dvl2, both full-length epsin 1 and ENTH-UIM constructs were sufficient to reduce Dvl2 polyubiquitination ( Fig. 7e ). For further confirmation, we used molecular modelling to identify critical residues within the ENTH (R8 and R25) and UIM (E184 and E198) domains of epsin 1 predicted to facilitate Dvl2 binding. Individual point mutations (R8A, R25G, E184A or E198G) and subsequent co-immunoprecipitation assays revealed significant reductions in epsin 1:Dvl2 binding ( Fig. 7f,g ) by all four mutants. To summarize our detailed domain-mapping data, epsin ENTH-UIM interacted with the C terminus of Dvl2 to impair Dvl2 polyubiquitination. Impaired polyubiquitination and increased stabilization of Dvl2 in the presence of epsins strongly suggested that epsins may competitively impede E3 ligase binding to the Dvl2 C terminus. Expressing ENTH-UIM or Dvl2 rescues tumour growth To directly test whether epsins facilitated canonical Wnt signalling by interacting with and stabilizing Dvl2, we subcloned the ENTH-UIM fragment into a lentiviral vector for stable infection and expression in mammalian cells. Epsin ENTH-UIM expression was confirmed after infection of HEK293T cells by qRT–PCR ( Fig. 8a ). Importantly, epsin ENTH-UIM fragment expression stabilized Dvl2 protein to levels similar to full-length epsin 1 overexpression ( Fig. 8b,c ). The lentiviral epsin ENTH-UIM vector was subsequently used to create stable epsin-depleted CMT-93 and HT-29 cells without or with expression of the ENTH-UIM fragment. Epsin depletion was confirmed by western blotting before lentiviral infection ( Fig. 8d,h ). Cells were subcutaneously implanted into severe combined immunodeficient (SCID) mice and tumour growth monitored. On the basis of our binding data, we hypothesized that the ENTH-UIM fragment would stabilize Dvl2, thus facilitating canonical Wnt signalling and tumour growth. Furthermore, by deleting the epsin 1 C terminus we limited the fragment’s clathrin-binding capabilities and, thus, its ability to modulate receptor internalization. Similar to our IEpC-iDKO mice, we determined that epsin depletion significantly hindered growth of both CMT-93 and HT-29 colon cancer cell xenografts ( Fig. 8e–g,i ). Expression of the epsin ENTH-UIM fragment was sufficient to recover tumour growth ( Fig. 8e–g,i ). In contrast, lentiviral expression of the C-terminal epsin DPW-NPF fragment failed to rescue tumour growth ( Fig. 8j ). These findings provided further evidence that epsins function to promote colon cancer growth, likely by stabilizing Dvl2. As proof, Dvl2 overexpression in epsin-deficient cells rescued Wnt signalling activation ( Fig. 3l ) and, likewise, overexpression of Dvl2 by retroviral infection in epsin-deficient CMT-93 colon cancer cells rescued tumour growth ( Fig. 8j ). In contrast, overexpression of active Notch, NICD, by retroviral infection did not rescue epsin-deficient tumour inhibition ( Fig. 8j ). The fact that either the ENTH-UIM fragment or Dvl2 expression, but not DPW-NPF fragment or NICD expression, was sufficient to recover tumour growth after epsin deficiency emphasized the importance of this novel mechanism for canonical Wnt signalling, independent of any role for epsin in Wnt receptor internalization or Notch signalling. 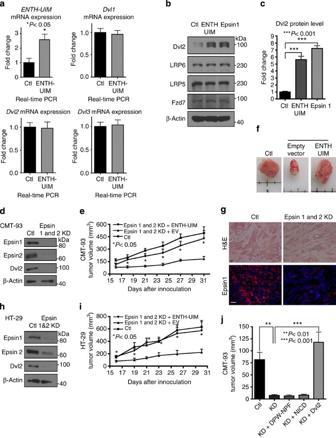Figure 8: The Epsin ENTH-UIM fragment was sufficient to recover tumour growth. (a) qRT–PCR analyses ofEpsin ENTH-UIM,Dvl1,Dvl2andDvl3mRNA expressions in HEK 293T cells infected with empty vector (EV)- or ENTH-UIM-expressing lentivirus,n=9. (b) Western blotting of HEK 293T cells infected with EV-, ENTH-UIM- or full-length epsin 1-expressing lentivirus. (c) Quantification of Dvl2 inb,n=6. (d) Western blotting of epsins 1 and 2 and Dvl2 in CMT-93 cells infected with EV or epsins 1 and 2 shRNA-expressing viruses,n=6. (e) Xenograft tumour volume analyses of control, epsin-depleted or epsin-depleted ENTH-UIM-expressing CMT-93 cells subcutaneously implanted in SCID mice,n=6. (f) Representative images at 31 days post implantation. (g) H&E and immunofluorescence staining of epsin 1 in representative CMT-93 xenograft tumours fromf. Scale bars, 50 μm. (h) Western blotting of epsins 1 and 2 and Dvl2 in HT-29 cells infected with EV or epsins 1 and 2 shRNA-expressing viruses,n=6. (i) Xenograft tumour volume analysis of control, epsin-depleted or epsin-depleted ENTH-UIM-expressing HT-29 cells subcutaneously implanted in SCID mice,n=6. (j) Final xenograft tumour volumes of control, epsin-depleted or epsin-depleted DPW-NPF-, NICD-myc- or Dvl2- expressing CMT-93 cells 18 days post-subcutaneous implantation in SCID mice,n=6. All statistical values were calculated using a Student’st-test;Pvalues are indicated. Error bars indicate the mean±s.e.m. Figure 8: The Epsin ENTH-UIM fragment was sufficient to recover tumour growth. ( a ) qRT–PCR analyses of Epsin ENTH-UIM , Dvl1 , Dvl2 and Dvl3 mRNA expressions in HEK 293T cells infected with empty vector (EV)- or ENTH-UIM-expressing lentivirus, n =9. ( b ) Western blotting of HEK 293T cells infected with EV-, ENTH-UIM- or full-length epsin 1-expressing lentivirus. ( c ) Quantification of Dvl2 in b , n =6. ( d ) Western blotting of epsins 1 and 2 and Dvl2 in CMT-93 cells infected with EV or epsins 1 and 2 shRNA-expressing viruses, n =6. ( e ) Xenograft tumour volume analyses of control, epsin-depleted or epsin-depleted ENTH-UIM-expressing CMT-93 cells subcutaneously implanted in SCID mice, n =6. ( f ) Representative images at 31 days post implantation. ( g ) H&E and immunofluorescence staining of epsin 1 in representative CMT-93 xenograft tumours from f . Scale bars, 50 μm. ( h ) Western blotting of epsins 1 and 2 and Dvl2 in HT-29 cells infected with EV or epsins 1 and 2 shRNA-expressing viruses, n =6. ( i ) Xenograft tumour volume analysis of control, epsin-depleted or epsin-depleted ENTH-UIM-expressing HT-29 cells subcutaneously implanted in SCID mice, n =6. ( j ) Final xenograft tumour volumes of control, epsin-depleted or epsin-depleted DPW-NPF-, NICD-myc- or Dvl2- expressing CMT-93 cells 18 days post-subcutaneous implantation in SCID mice, n =6. All statistical values were calculated using a Student’s t -test; P values are indicated. Error bars indicate the mean±s.e.m. Full size image Epsin is upregulated in mouse colon cancer in vivo To confirm that epsins were upregulated in mouse colon cancer, and that this upregulation correlated with upregulated Dvl2 and Wnt receptor expression, we used immunofluorescence to stain normal and tumorous colon tissue sections from control and AOM/DSS-treated WT mice. We found that epsin 1, Dvl2, Fzd7 and Fzd8 were upregulated in mouse colon tumours, compared with normal tissues ( Fig. 9a–c ). Furthermore, and similar to human colon cancer ( Fig. 1 ), these expression levels correlated strongly with tumour severity such that expressions in malignant adenocarcinomas were higher than benign adenomas, which were in turn higher than normal tissues ( Fig. 9d–g ). We focused our staining on epsin 1, Dvl2 and Fzd7 after determining that epsin 1 mRNA expression was dominant over epsin 2 ( Fig. 9h ), Dvl2 over Dvl1 or Dvl3 ( Fig. 5c ) and Fzd7 over Fzd8 ( Fig. 9i ) in mouse CMT-93 cells. 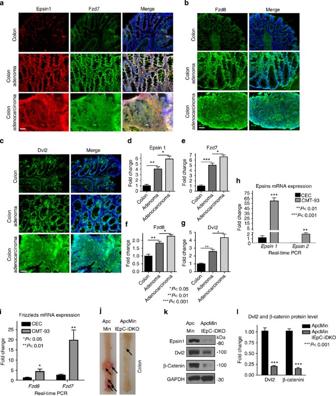Figure 9: Epsin 1, Dvl2 and Wnt receptors were upregulated in mouse colon cancer. (a–c) Epsin 1 and Fzd7 (a), Fzd8 (b) and Dvl2 (c) were analysed by immunofluorescence staining of peripheral normal, adenoma and adenocarcinoma colon tissues from control and AOM/DSS-treated WT mice. Scale bar:, 50 μm. (d–g) Quantifications of epsin 1 (d), Fzd7 (e), Fzd8 (f) and Dvl2 (g) staining ina–c,n=11. (h,i) qRT–PCR analyses ofepsin 1andepsin 2(h) orFzd7andFzd8(i) mRNA expressions in WT CECs and the CMT-93 mouse colon cancer cell line,n=9. (j) Representative image of longitudinally cut colons and rectums of ApcMinand ApcMin/IEpC-DKO mice killed at 20 weeks of age; arrows indicate tumours in colon and rectal regions,n=11. (k) Western blotting of epsin 1, Dvl2 and β-catenin in the colon epithelia from ApcMinand ApcMin/IEpC-DKO mice. (l) Quantification of Dvl2 and β-catenin ink,n=6. All statistical values were calculated using a Student’st-test;Pvalues are indicated. Error bars indicate the mean±s.e.m. Figure 9: Epsin 1, Dvl2 and Wnt receptors were upregulated in mouse colon cancer. ( a – c ) Epsin 1 and Fzd7 ( a ), Fzd8 ( b ) and Dvl2 ( c ) were analysed by immunofluorescence staining of peripheral normal, adenoma and adenocarcinoma colon tissues from control and AOM/DSS-treated WT mice. Scale bar:, 50 μm. ( d – g ) Quantifications of epsin 1 ( d ), Fzd7 ( e ), Fzd8 ( f ) and Dvl2 ( g ) staining in a – c , n =11. ( h , i ) qRT–PCR analyses of epsin 1 and epsin 2 ( h ) or Fzd7 and Fzd8 ( i ) mRNA expressions in WT CECs and the CMT-93 mouse colon cancer cell line, n =9. ( j ) Representative image of longitudinally cut colons and rectums of Apc Min and Apc Min /IEpC-DKO mice killed at 20 weeks of age; arrows indicate tumours in colon and rectal regions, n =11. ( k ) Western blotting of epsin 1, Dvl2 and β-catenin in the colon epithelia from Apc Min and Apc Min /IEpC-DKO mice. ( l ) Quantification of Dvl2 and β-catenin in k , n =6. All statistical values were calculated using a Student’s t -test; P values are indicated. Error bars indicate the mean±s.e.m. Full size image Epsin loss reduces tumour rate in Apc Min colon cancer model Familial adenomatous polyposis (FAP), a hereditary human intestinal cancer syndrome, as well as many forms of sporadic human colon cancers, are caused by genetic mutations that promote β-catenin stabilization downstream of Wnt receptor activation and Dvl2 (refs 3 , 14 , 22 , 42 , 58 ). Given the importance of these downstream alterations, it remained unclear what implications epsins’ novel role in stabilizing Dvl2, and the potential disruption of this interaction, would have on genetic models of colon cancer. To investigate, we engineered an epsin-deficient genetic model for colon cancer by crossing our Epn1 fl/fl ;Epn2 −/− ; Villin-ER T2 Cre mice with the well-characterized FAP-model Apc Min mice, which are heterozygous for a truncation mutation of the Apc gene [59] . Postnatal epsin 1 deletion was induced as described above. Tumour incidence was evaluated in WT or Apc Min /IEpC-iDKO colons isolated 20 weeks after tamoxifen-induced epsin deletion. Epsin deficiency was found to protect against tumour development in the colons ( Fig. 9j ) and small intestines ( Supplementary Fig. 3 ) of Apc Min /IEpC-iDKO mice. Consistent with epsins’ role in Dvl2 stabilization, loss of epsins in Apc Min mice significantly reduced the Dvl2 protein ( Fig. 9k,l ). Reduced Dvl2 protein directly correlated with significant loss of β-catenin ( Fig. 9k,l ), despite the genetic destabilization of the β-catenin destruction complex. This phenotype closely mimicked the phenotype of the previously reported tumour-resistant APC Min /Dvl2 − / − mice [22] . The similarities of our APC Min /IEpc-iDKO mice in which epsin loss destabilized Dvl2 to prevent colon cancer and the tumour-resistant phenotype after genetic ablation of Dvl2 (APC Min /Dvl2 − / − mice) provided strong evidence that β-catenin activation can be modulated, despite alterations of the β-catenin destruction complex. Therefore, we propose that Dvl2 stability, modulated in part by epsins, is critical for the aberrant Wnt-dependent stabilization of β-catenin responsible for excessive tumour cell proliferation and colon cancer development. Furthermore, our finding emphasized the potential usefulness of epsin inhibition in preventing FAP by destabilizing Dvl2 and β-catenin. We previously reported that epsins, specifically endothelial epsins, played a critical role in regulating the tumour microenvironment to promote cancer progression [37] , [38] . However, epsins are also reportedly upregulated in tumours; however, the critical role for this upregulation within a given tumour cell type was still unknown [36] , [39] , [40] , [41] . In this study, we revealed that epsins were significantly upregulated in both human and mouse colon cancer. Further, we discovered a novel role for epsins in the regulation of canonical Wnt signalling independent of its classical role as an endocytic adaptor. As discussed previously, deregulated canonical Wnt signalling is an established pathway involved in colon cancer development and progression [1] , [2] , [14] . Although several genetic mutations within β-catenin and its destruction complex are known to cause deregulation, other mechanisms of regulation including Wnt receptor expression, activation and internalization have also been implicated [4] , [12] , [13] , [16] , [18] , [19] . Consistently, we found that both human and mouse colon cancers exhibited parallel upregulation of epsins, Dvl2 and Fzd ( Figs 1 and 9 ). Furthermore, epsin expression levels tightly correlated with the aggressiveness of the tumour. These findings, in combination with the fact that loss of intestinal epithelial epsins inhibited both canonical Wnt signalling and colon cancer progression ( Figs 2 , 3 and 9 ), provided strong evidence suggesting that intestinal epithelial epsins play an important role in regulating Wnt signalling; however, given epsin’s classic role as an endocytic adaptor, we were surprised to find that, while epsins were necessary for canonical Wnt signalling activation and colon cancer development, they were dispensable for internalization-dependent activation of the Wnt receptors ( Fig. 4e,f ). We had already determined via the luciferase assay that loss of epsins inhibited canonical Wnt signalling upstream of β-catenin stabilization and was dependent in part on Dvl2 ( Fig.3k,l ). Our internalization data further indicated that the inhibitory effect was downstream of receptor internalization. Given that Dvl2 is the signalling molecule that connects Wnt receptor activation with β-catenin stabilization through regulated disassembly of the destruction complex, we investigated the effects of epsin deficiency on Dvl2 (refs 23 , 24 ). Our discovery that epsins constitutively associated with Dvl2 ( Fig. 4a ), that loss of epsins significantly diminished Dvl2 protein levels ( Fig 5l ) and that Dvl2 overexpression rescued the epsin-deficient phenotype ( Figs 3l and 8j ) provided a much needed explanation for how epsin deficiency abolished canonical Wnt signalling. For the first time, we have identified a novel role for epsin as a cytosolic chaperone protein, a role completely independent of its classical role as a membrane-associated endocytic adaptor. In light of our extensive mechanistic binding analyses, we propose a model in which epsin interacts constitutively with the C terminus of Dvl2 via its ENTH and UIM domains, presumably prohibiting E3 ligase binding, and thus reducing Dvl2 ubiquitination and degradation ( Fig. 10 ). The epsin:Dvl2 complex is subsequently recruited to the Wnt receptor complex, thus explaining the Wnt-dependent association between epsin and the Wnt receptors. As such, we propose that epsins are critical regulators for Wnt signalling activation and colon cancer progression by protecting Dvl2 from proteasomal degradation ( Fig. 10 ). Our proposed mechanism explains how the loss of epsins leads to the loss of Dvl2 and decreased tumour progression in IEpC-iDKO mice, and further provides a potential explanation for why epsins and Dvl2 are correspondingly upregulated in both mouse and human colon cancers. 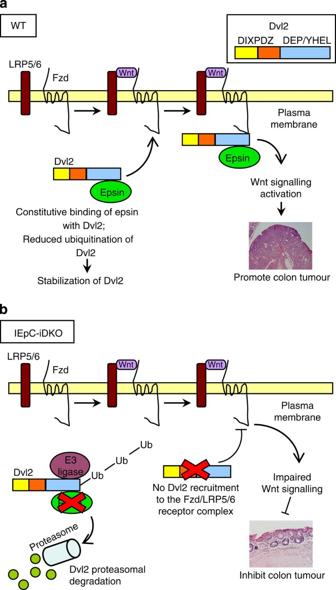Figure 10: Schematic model of the interaction between epsin and Dvl2. (a) Epsins bind to the C terminus of Dvl2 independent of Wnt stimulation, thus protecting Dvl2 from E3 ligase-mediated polyubiquitination and degradation. Wnt stimulation, and subsequent activation of the Fzd:LRP receptor complex, recruits epsin-associated Dvl2 to the complex. Complex-associated epsins may further stabilize the complex and promote its internalization, a necessary event for Wnt signalling, through interactions between epsin UIM and the Wnt receptors. Activated Wnt signalling promotes colon epithelial tumour progression. (b) Epsin deficiency reduces Dvl2 stability resulting in reduced Wnt-dependent signalling activation. Impaired Wnt signalling activation results in reduced colon epithelial tumour progression. Figure 10: Schematic model of the interaction between epsin and Dvl2. ( a ) Epsins bind to the C terminus of Dvl2 independent of Wnt stimulation, thus protecting Dvl2 from E3 ligase-mediated polyubiquitination and degradation. Wnt stimulation, and subsequent activation of the Fzd:LRP receptor complex, recruits epsin-associated Dvl2 to the complex. Complex-associated epsins may further stabilize the complex and promote its internalization, a necessary event for Wnt signalling, through interactions between epsin UIM and the Wnt receptors. Activated Wnt signalling promotes colon epithelial tumour progression. ( b ) Epsin deficiency reduces Dvl2 stability resulting in reduced Wnt-dependent signalling activation. Impaired Wnt signalling activation results in reduced colon epithelial tumour progression. Full size image Since its original discovery in 1998 (ref. 30 ), epsins have been implicated in several proliferative signalling pathways including Notch [34] , [37] , [38] , [50] , [60] . In Drosophila, Notch and Wnt signalling pathways crosstalk to ensure proper development [60] . Notably, epsins (liquid facets) play a pivotal role in Drosophila development through the regulation of Notch signalling, but do not appear to alter Wnt signalling as evident by the lack of a wingless phenotype when epsins were depleted [34] , [60] , [61] , [62] . Our data however strongly indicate that epsin is a critical regulator for Wnt signalling in mammalian vertebrates because in our novel IEpC-iDKO mice Wnt signalling is dramatically impaired by loss of epsins. Nonetheless, it remained a possibility that intestinal epithelial epsin loss also impaired tumour growth by modulating Notch signalling, given the previously determined role of epsins as promoters of Notch signalling [63] , [64] , [65] , [66] . However, in colon cancer, Notch signalling counteracts Wnt signalling resulting in reduced expression of β-catenin target genes and impaired colon cancer cell proliferation [67] . The fact that epsin depletion in the intestinal epithelial cells significantly impaired, instead of promoted, colon cancer progression supposedly produced by Notch signalling inhibition suggested that, at least in colon cancer, epsin-mediated Notch signalling does not play a significant role in regulating cancer progression. This is further supported by the fact that expression of the active form of Notch, NICD, did not rescue tumour growth in our epsin-deficient subcutaneous colon cancer model ( Fig. 8j ). In our final observations, we found that, in addition to colitis-induced colon cancer, intestinal epithelial epsin deficiency also sufficiently protected against colon cancer development in the well-characterized genetic Apc Min model of FAP. These findings mimicked those previously reported in Apc Min /Dvl2 − / − mice including reduced β-catenin activity, canonical Wnt signalling and colon cancer development despite genetic destabilization of the β-catenin destruction complex [22] . This previous report also determined that loss of Dvl2 protected against tumour development by reducing canonical Wnt signalling in Apc Min /Dvl2 − / − mice. Although the Apc Min mutation promotes constitutive β-catenin stabilization downstream of Dvl2 stabilization and Wnt-dependent recruitment, our discovery that epsin loss destabilized both Dvl2 and β-catenin despite, the mutated destruction complex, emphasized the importance of epsin-mediated stabilization of Dvl2 to Wnt signalling, intestinal epithelial cell proliferation and colon cancer progression. Furthermore, this finding supports a potential use for targeted inhibition of epsins in the therapeutic treatment of a variety of colon cancers despite the fact that a significant percentage of them results from genetic mutations that directly stabilize β-catenin through inhibition of the destruction complex. A significant amount of effort was previously spent on developing anti-Wnt therapies to combat cancer but progress has been limited due to high toxicity, minimal efficacy and/or off-target effects [68] , [69] . Our findings suggest that targeting epsins represents a potential novel strategy to combat colon cancer and provides hope for patients who are resistant or unresponsive to current anticolon cancer therapies. Generation of conditional IEpC-iDKO and APC Min mice We reported a strategy to generate an epsin 1 and 2 global DKO mouse model [34] . We used a similar strategy with modifications to create a conditional knockout of epsin 1 ( Epn1 fl/fl mice) [34] , [37] . Epn1 fl/fl mice were mated with Epn2 −/− null mice to generate Epn1 fl/fl ;Epn2 −/− mice. Tamoxifen-inducible IEpC-specific DKO (IEpC-iDKO) mice were obtained by crossing Epn1 fl/fl ;Epn2 −/− mice with Villin-ER T2 Cre deleter mice that express Cre recombinase specifically in the IEpCs [44] . To induce postnatal deletion of IEpC epsin 1, we administered 5 mg kg −1 (body weight) of 4-hydroxytamoxifen by intraperitoneal-injection into 10-week-old WT or Epn1 fl/fl ;Epn2 −/− ;Villin-ER T2 mice every second day for 2 weeks. To generate the Apc Min /IEpC-iDKO mice, we crossed our Epn1 fl/fl ;Epn2 −/− ;Villin-ER T2 mice with Apc Min mice purchased from Jackson Laboratories. All vertebrate procedures were performed in accordance with the Guide for the Care and Use of Laboratory Animals and were approved by the Institutional Animal Care and Use Committee at Oklahoma Medical Research Foundation. Antibodies and reagents Unless specified otherwise, common laboratory chemicals and reagents were from either Sigma-Aldrich or Fisher Scientific. Media and additives for cell culture were from Gibco. The reagents and materials for RNA isolation, qRT–PCR, transfection reagents, primers and siRNA were from Invitrogen. The Dual-Luciferase Reporter Assay Kit was from Promega. The QuikChange II Site-Directed Mutagenesis Kit was from Agilent Technologies. BrdU, 4-hydroxytamoxifen and AOM were from Sigma-Aldrich. DSS was from MP Chemicals Inc. Recombinant mouse and human Wnt3a were from R&D systems. GSK3-βi (CHIR-99021) was from Selleckchem. MG132 was from Calbiochem. Polyclonal rabbit antibodies for epsin 1 (1:2,000 western blotting dilution) and epsin 2 (1:4,000 western blotting dilution) were obtained as described [30] , [31] . Anti-Epsin 1 (1:1,000 western blotting dilution; 1:200 immunofluorescence dilution; 1:200 immunoprecipitation dilution), -glyceraldehyde-3-phoshate dehydrogenase (1:3,000 western blotting dilution), -LRP5 (1:500 western blotting dilution), -LRP6 (1:500 western blotting dilution), -Fzd7 (1:500 western blotting dilution; 1:50 immunofluorescence dilution), -Fzd8 (1:500 western blotting dilution; 1:50 immunofluorescence dilution), -cMyc (1:1,000 western blotting dilution) and -cyclin D1 (1:1,000 western blotting dilution) antibodies were from Santa Cruz Biotechnologies; anti-β-catenin antibody (1:3,000 western blotting dilution; 1:100 immunohistochemistry) was from BD; anti-Dvl2 (1:2,000 western blotting dilution; 1:100 immunofluorescence dilution; 1:200 immunoprecipitation dilution) and anti-phospho-LRP6 (Ser1490; 1:1,000 western blotting dilution) antibodies were from Cell Signaling Technology; anti-β-actin antibody (1:3,000 western blotting dilution) was from Invitrogen; anti-HA antibody (1:2,000 western blotting dilution; 1:200 immunoprecipitation dilution) was from Covance; anti-Flag antibody (1:2,000 western blotting dilution; 1:200 immunoprecipitation dilution) was from Sigma-Aldrich. Colitis-induced mouse colon cancer model Colitis-inducible colon cancer mouse model was created as described [45] . Briefly, 12- to 13-week-old WT or IEpC-iDKO mice were given a single intraperitoneal-injection of AOM (10 mg kg − 1 body weight). One week after injection, mice received 2% DSS in drinking water for 7 days followed by no further treatment. Mice were killed 20 weeks after the initial AOM injection. The colons and rectums were cut open longitudinally and examined for tumours. The number and size of tumours were recorded. In vivo colon tumour xenograft assay Control, epsin-deficient or epsin-deficient ENTH-UIM-, DPW-NPF-, Dvl2- or NICD-expressing CMT-93 or HT-29 colon cancer cells were implanted subcutaneously (5 × 10 6 cells per injection) in 12-week old SCID mice. We recognized tumours more than 2 mm in diameter as positive. Tumour growth was monitored by measuring tumour size using a digital caliper. Tumour volumes were calculated on the basis of the formula: 0.5326 (length [mm] × width 2 [mm 2 ]). Tumours were harvested, photographed, embedded and processed for staining as described below. Histological examination AccuMax human tissue microarray test slides of 12 colon adenomas and adenocarcinomas with corresponding non-neoplastic tissues (A713 VIII) were obtained from ISU ABXIS. Mouse tissues were harvested, fixed in 10% formalin and embedded in paraffin. All sections were stained with H&E according to the standard procedures or by immunohistochemistry or immunofluorescence as described below. In vivo BrdU labelling Mice were intraperitoneally injected with BrdU (100 mg kg − 1 body weight). Colon tumours from AOM/DSS-treated mice were carefully harvested 3 h post injection, fixed in 10% formalin and paraffin-embedded. Paraffin sections were deparaffinized with xylene and alcohol series. After inactivation of endogenous peroxidase with 0.3% hydrogen peroxide and blocking with normal blocking serum, the sections were labelled using a mouse anti-BrdU antibody. After washing, the sections were incubated with biotinylated secondary antibody in the Vectastain Elite ABC staining kit (Vector Laboratories) for 1 h at room temperature, followed by treatment with the ABC reagent for 30 min. Aminoethyl carbazole was used as the peroxidase substrate. Sections were washed, counterstained with haematoxylin, mounted and photomicrographs were obtained. Immunohistochemistry and immunofluorescence staining For IHC staining: Sections were deparaffinized with xylene and alcohol series. After inactivation of endogenous peroxidase with 0.3% hydrogen peroxide and blocking with normal blocking serum, the sections were incubated with anti-β-catenin antibody overnight at 4 °C. After washing, the sections were incubated with biotinylated secondary antibody (1:500) in the Vectastain Elite ABC staining kit (Vector Laboratories) for 1 h at room temperature, followed by treatment with the ABC reagent for 30 min. Aminoethyl carbazole was used as the peroxidase substrate. Sections were then washed, counterstained with haematoxylin, mounted and photomicrographs were obtained. Tissues stained with omission of primary antibody were captured using the same settings and used as negative controls. For immunofluorescence staining: Cryosections were blocked as described above and then incubated with primary antibody overnight at 4 °C, followed by incubation with the respective secondary antibodies conjugated to fluorescent labels (Alexa Flour 594 or 488; 1:500; Invitrogen) for 1 h at room temperature. Slides were washed in PBS, stained with 4',6-diamidino-2-phenylindole (100 ng ml − 1 ), mounted and immunofluorescence images were obtained using Olympus Fluorescence Microscopy equipped with the Slidebook 5.0 analysis software [37] . Tissues stained with omission of primary antibody were captured using the same settings and were used as negative controls. Isolation of adult mouse colon epithelium Colons of adult mice were isolated and the epithelium extracted by shaking the chopped colon in Dulbecco’s PBS containing 30 mM EDTA, 10% fetal bovine serum (FBS), 1 mM dithiothreitol (DTT), pH 8.0 at 4 °C for 30–40 min followed by centrifugation at 900 × g at 4 °C for 10 min. Colon epithelia were used to confirm epsin KD via western blotting and to detect transcription of Wnt pathway downstream genes via qRT–PCR. Cell culture Isolation and culture of primary mouse CECs from 4- to 6-day-old WT or Epn1 fl/fl ;Epn2 −/− ; Villin-ER T2 Cre pups was performed as described [70] . Briefly, colons were harvested, split longitudinally, diced into very small fragments and washed in PBS–Glucose (PBS supplemented with 2% glucose and 1% penicillin/streptomycin). After excess fluid removal, colon fragments were digested for 1 h at 37 °C in PBS–Glucose supplemented with 100 μg ml − 1 Dispase type II and 2 mg ml − 1 Crude Collagenase type I. After crypt isolation was confirmed by microscopy, digestion enzymes were neutralized in Dulbecco’s modified Eagle’s medium (DMEM)-sorbitol (DMEM supplemented with 5% fetal calf serum and 2% sorbitol). Supernatant containing crypts was obtained after a series of 1-min gravity sedimentation cycles. Single-cell contaminants were removed by centrifugation at 300 r.p.m. for 3 min. After isolation, colon epithelial progenitor cell-containing crypt aggregates were seeded on culture dishes pre-coated with 0.2% gelatin and cultured at 37 °C with 5% CO 2 in high-glucose DMEM supplemented with 10% FBS, 0.25 IU ml − 1 insulin, 20 ng ml − 1 epidermal growth factor, 50 μg ml − 1 heparin and 1% penicillin/streptomycin. After 2–3 days, CECs were treated with 5 μM 4-hydroxytamoxifen for 72 h to induce epsin 1 deletion. Freshly isolated primary CECs were used for all experiments without further passage. The HT-29 (human colorectal adenocarcinoma cell line, ATCC no. HTB-38) and CMT-93 (mouse rectum carcinoma cell line, ATCC no. CCL-223) cell lines were cultured at 37 °C with 5% CO 2 in high-glucose DMEM supplemented with 10% FBS and 1% penicillin/streptomycin. The HEK 293T cell line (ATCC no. CRL-11268) was cultured at 37 °C with 5% CO 2 in high-glucose DMEM supplemented with 10% FBS and 1% penicillin/streptomycin. RNA interference HT-29 cells were transfected by RNAiMAX according to the manufacturer’s instructions with siRNA duplexes of scrambled or human epsin 1 (UGCUCUUCUCGGCUCAAACUAAGGG) and epsin 2 (AAAUCCAACAGCGUAGUCUGCUGUG), designed using Ambion Silencer Select Predesigned siRNAs (Invitrogen). At 48 h post transfection, cells were processed for western blotting. Plasmids and transfection Flag-tagged Dvl2, unphosphorylatable β-catenin, HA-ubiquitin and NICD-myc plasmids were obtained from Addgene. Retroviral pLEX expression system was from Thermoscientific. Epsin 1 and epsin 1 ΔUIM plasmids and lentiviral pLL3.7 RNA interference vectors encoding epsin 1 and 2 short hairpin RNA (shRNA) were described previously [29] . All remaining truncation and single-domain constructs were generated using standard subcloning procedures. Epsin 1 point mutations were made using the QuikChange Site-Directed Mutagenesis Kit as per the manufacturer’s instruction. Epsin 1 point mutations were predicted using three-dimensional modelling by PEP-FOLD ( http://bioserv.rpbs.univ-paris-diderot.fr/PEP-FOLD ) and ClusPro ( http://cluspro.bu.edu ). Cloning and mutagenesis primers are available upon request. HEK 293T cells were transfected using Lipofectamine 2000 as instructed by the manufacturer. Lentiviral production was accomplished by transfecting Phoenix ECO cells (ATCC no. CRL-3214) using Lipofectamine 2000. Viruses were harvested 48 h post transfection. RNA isolation and quantitative real-time PCR Total RNA was extracted using the Trizol reagent. One microgram of total RNA was treated with 1 U RNase-free DNase I to eliminate genomic DNA. The first-strand cDNA was synthesized using the SuperScript III First-Strand Synthesis SuperMix. An aliquot of 1 μl of the product was subjected to qRT–PCR in a 7300 Real-Time PCR System (Applied Biosystems) using SYBR Green PCR Master Mix reagent as the detector. PCR amplification was performed in triplicate on 96-well optical reaction plates and replicated in three independent experiments. Gel electrophoresis and melting curve analyses were performed to confirm correct PCR product sizes and absence of nonspecific bands. Immunoprecipitation and western blotting For Wnt signalling assays, CECs that had been starved overnight in a serum-free medium were treated with 100 ng ml − 1 of Wnt3a for 0, 5, 15 or 30 min or 1, 2, 4, 6 or 8 h at 37 °C, and then washed twice with ice-cold PBS, lysed in Laemmli buffer and processed for western blotting. For the MG132 experiments, cells were serum-starved overnight in DMEM, pretreated for 4 h with 10 μM MG132, stimulated without or with Wnt3a as indicated and then prepared for western blotting as described above. For immunoprecipitation, transfected HEK 293T cells were lysed with RIPA buffer (1% Triton X-100, 0.1% SDS, 0.5% sodium deoxycholic acid, 5 mM tetrasodium pyrophosphate, 50 mM sodium fluoride, 5 mM EDTA, 150 mM NaCl, 25 mM Tris, pH 7.5, 4 mM Na 3 VO 4 , 5 mM N-ethylmaleimide and protease inhibitor cocktail). For Dvl2 ubiquitination experiments, cells were lysed using one volume of denaturing buffer (1% SDS in 50 mM Tris, pH 7.5) and boiled for 10 min at 100 °C to denature protein complexes. Lysates were re-natured using nine volumes of ice-cold RIPA buffer and then prepared for immunoprecipitation as follows. Cell lysates were pre-cleared with mouse IgG and protein G Sepharose beads for 2 h at 4 °C followed by incubation with antibodies against epsin 1, Dvl2, Flag or HA for 4 h at 4 °C. For negative controls, equal concentration of mouse IgG was added instead of specific antibodies. Precipitated proteins were eluted from beads using 2% SDS in 50 mM Tris, pH 7.5 and diluted 1:20 with RIPA buffer followed by western blotting. Proteins were resolved by SDS–PAGE (7.5% acrylamide) followed by electroblotting to a polyvinylidene difluoride membrane and blocking with 3% milk (weight per volume). Primary antibodies were incubated at 4 °C overnight, followed by incubation at room temperature with the respective horseradish peroxidase-conjugated secondary antibodies (1:2,000) for 1 h. The immunoreactive proteins were detected by enhanced chemiluminescence with autoradiography. Western blots were quantified using the NIH ImageJ software. Uncropped images of the western blots depicted in the main figures are available in Supplementary Fig. 4 . Luciferase reporter assay HEK 293T cells were serum-starved overnight and co-transfected with either TOPflash (containing TCF-binding sites) or FOPflash (mutant, inactive TCF-binding sites) luciferase expression vectors and with Renilla luciferase vector (control) using Lipofectamine 2000 (ref. 54 ). Sixteen hours post transfection, cells were incubated with recombinant human Wnt3a and/or CHIR-99021, an inhibitor of GSK3-β (GSK3-βi). After 8 h, luciferase activity in total cell lysates was measured using Dual-Luciferase Reporter Assay Kit (Promega) and was normalized for transfection efficiency via dividing by the Renilla luciferase activity. The TOP/FOP ratio was used as a quantitative measure of β-catenin-mediated TCF4 activity. Internalization of biotinylated LRP6 Primary CECs were serum-starved overnight and incubated with 1 nM cleavable EZ-Link Sulfo-NHS-S-S-Biotin dissolved in cold PBS at 4 °C for 30 min with gentle shaking. Cells were washed with cold PBS plus 50 mM glycine to stop biotinylation. Cells were then changed to warm media with 100 ng ml − 1 Wnt3a and incubated at 37 °C for 0, 5, 15 or 30 min. Remaining surface biotin was cleaved by incubating with cleavage buffer (23 mM NaH 2 PO 4 , 27 mM Na 2 HPO 4 , 75 mM NaCl, 1% BSA, 10 mM EDTA, pH 8.0 and 50 mM DTT) three times for 15 min each at 4 °C with gentle shaking. Cells were lysed in RIPA buffer and processed for streptavidin bead pull-down. Pull-downs were separated by SDS–PAGE and analysed by western blotting. Endocytosed LRP6 was visualized by western blotting using the anti-LRP6 antibody. Statistical analysis We used 11 animals in all groups to detect at the 0.05 significance level with power of 0.80–0.90, an effect size of 1.55–1.65 s.d. units with the two-tailed Student’s t -test. Immunoprecipitation, western blotting, IF and IHC staining, and luciferase reporter assays were replicated six to eight times to achieve similar 0.05 significance using two-tailed Student’s t -tests. Quantitative RT–PCR was carried out in triplicate and replicated three times to achieve 0.05 significance using two-tailed Student’s t -test. All data are represented as the mean+s.e.m and the P values were indicated. A P value of less than 0.05 was considered statistically significant. How to cite this article: Chang, B. et al. Epsin is required for dishevelled stability and Wnt signalling activation in colon cancer development. Nat. Commun. 6:6380 doi: 10.1038/ncomms7380 (2015).